Screening of DUB activity and specificity by MALDI-TOF mass spectrometry Deubiquitylases (DUBs) are key regulators of the ubiquitin system which cleave ubiquitin moieties from proteins and polyubiquitin chains. Several DUBs have been implicated in various diseases and are attractive drug targets. We have developed a sensitive and fast assay to quantify in vitro DUB enzyme activity using matrix-assisted laser desorption/ionization time-of-flight (MALDI-TOF) mass spectrometry. Unlike other current assays, this method uses unmodified substrates, such as diubiquitin topoisomers. By analysing 42 human DUBs against all diubiquitin topoisomers we provide an extensive characterization of DUB activity and specificity. Our results confirm the high specificity of many members of the OTU and JAB/MPN/Mov34 metalloenzyme DUB families and highlight that all USPs tested display low linkage selectivity. We also demonstrate that this assay can be deployed to assess the potency and specificity of DUB inhibitors by profiling 11 compounds against a panel of 32 DUBs. Posttranslational modifications with ubiquitin control almost every process in cells. Ubiquitylation is facilitated by ubiquitin-activating (E1s), ubiquitin-conjugating (E2s) and ubiquitin ligase enzymes (E3s). Ubiquitin can be attached to substrate proteins as a single moiety or in the form of polymeric chains in which successive ubiquitin molecules are connected through specific isopeptide bonds. These bonds can be formed on any of the eight primary amines of the ubiquitin molecule (linear/amino (N) terminus/M1, K6, K11, K27, K29, K33, K48 and K63) and thus can achieve a remarkable complexity, termed the ubiquitin code [1] , in which the different chain topologies serve distinct signalling functions [2] . Ubiquitylation is reversible by specific cleavage through deubiquitylases (DUBs), of which about 90 have been identified in the human genome [3] . DUBs have been divided into five subclasses: ubiquitin carboxy (C)-terminal hydrolases (UCHs), ubiquitin-specific proteases (USPs), Machado–Joseph disease protein domain proteases (MJDs), ovarian tumour proteases (OTUs) and JAB/MPN/Mov34 metalloenzyme (JAMM) domain proteases [3] , [4] , [5] . UCHs, USPs, OTUs and MJDs function as papain-like cysteine proteases, whereas JAMMs are zinc-dependent metalloproteases [6] . A sixth family of DUBs, monocyte chemotactic protein induced proteases has recently been proposed, but little is known about this family so far [4] , [6] . DUBs have an essential role in ubiquitin homeostasis by catalysing the editing and disassembly of polyubiquitin chains [4] . Furthermore, DUBs also perform signalling functions by the regulatory deubiquitylation of target proteins [3] controlling proteasome-dependent protein degradation [7] , endocytosis [8] , DNA repair [9] and kinase activation [10] , [11] . Not surprisingly, DUBs have been implicated in a number of diseases such as cancer [12] , [13] , [14] , [15] , [16] , [17] , inflammation [10] , [18] , neurodegeneration/Parkinson’s disease [19] , [20] , [21] and, due to their potentially drugable active sites, are considered attractive drug targets [22] . Several chemical probes, such as Ub-vinyl methylester, Ub-vinyl sulphone [23] , branched and ubiquitin isopeptide activity-based probes [24] or diubiquitin activity probes [25] have been developed to explore the catalytic properties of DUBs. To screen for DUB inhibitors, current methods make use of non-physiological substrates including linear fusion of ubiquitin to a reporter protein such as phospholipase 2 or yellow fluorescent protein in a Fluorescent Resonance Energy Transfer assay format [26] , [27] . Moreover, fusions of fluorogenic reporters such as Rhodamine110 (ref. 28 ) or 7-amino-4-methylcoumarin [29] to the C-terminal glycine of ubiquitin are also widely deployed. However, these substrates are not suitable for assessing the linkage specificity of DUBs. Furthermore, as these are artificial substrates that do not contain physiological isopeptide bonds, screening assays using these substrates could potentially identify compounds that might not inhibit the deubiquitylation of physiological substrates. To circumvent these issues it is possible to undertake DUB assays with more physiologically related diubiquitin molecules [30] . However these assays are currently performed using low-throughput SDS–PAGE methodology and require relatively large amounts of enzymes (0.01–1 μg per assay) and substrates (typically up to 4 μg of substrate per assay) [31] . Matrix-assisted laser desorption/ionization (MALDI) time-of-flight (TOF) mass spectrometry (MS) [32] , [33] has in the past been successfully applied to quantify low molecular weight products of enzymes [34] or amyloid-beta peptides produced by gamma-secretase [35] . Here, we present a novel screening method to assay DUB activity and specificity using unmodified diubiquitin isomer substrates. We employ quantitative MALDI-TOF MS using 15 N-labelled ubiquitin and achieve high sensitivity, reproducibility and robustness. We analyse the specificity of 42 human DUBs and characterize the potency and selectivity of 11 DUB inhibitors against a panel of 32 DUBs. Our data represent an important resource for the scientific community and establish the applicability of the MALDI-TOF DUB assay in DUB inhibitor screening and selectivity assessment. MALDI-TOF DUB assay to assess DUB activity and specificity We have developed a fast and sensitive assay to analyse in vitro activity and specificity of DUBs by MALDI-TOF mass spectrometry, termed the MALDI-TOF DUB assay. In this assay, we quantitate the amount of monoubiquitin generated by the in vitro cleavage of specific diubiquitin topoisomers by DUBs ( Fig. 1a ). The DUB reaction consists of recombinant DUB (0.1–1,000 ng), diubiquitin (typically 125 ng, or 7,300 fmol) in 40 mM Tris–HCl pH 7.5, 5 mM dithiothreitol (DTT) and bovine serum albumin (BSA) carrier (0.25 μg) in a total volume of 5 μl. Reactions are undertaken for 1 h at 30 °C and terminated by addition of 1 μl of 10% (v/v) trifluoroacetic acid. Aliquots (2 μl) of each sample are spiked with 2 μl (1,000 fmol) of 15 N-labelled ubiquitin (average mass 8,666.55 Da), whose concentration was established by amino acid analysis, to serve as an internal standard for ubiquitin quantitation. A further 2 μl of 15.2 mg ml −1 2,5-dihydroxyacetophenone (DHAP) matrix and 2 μl of 2% (v/v) trifluoroacetic acid are added and 0.5 μl of the resultant mixture is then spotted onto a 1,536 microtiter plate MALDI anchor target. The samples are analysed by high mass accuracy MALDI-TOF MS in reflector positive ion mode on an UltrafleXtreme (Bruker Daltonics) mass spectrometer. 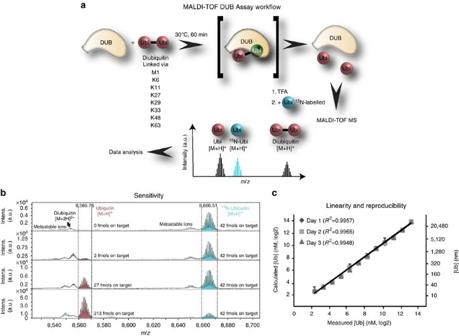Figure 1: The MALDI-TOF DUB assay. (a) Workflow of the MALDI-TOF DUB assay. Each of the 42 DUBs was incubated with all eight diubiquitin isomers individually (M1, K6, K11, K27, K29, K33, K48 and K63) for 60 min at 30 °C. The reaction was stopped with 2% TFA and mixed 1:1 with 0.5 μM15N-ubiquitin which serves as an internal standard. Subsequently, the analyte is mixed with 2,5 DHAP matrix and spotted onto a 1,536 AnchorChip MALDI target (Bruker Daltonics). Data analysis is performed using FlexAnalysis (Bruker Daltonics). (b) The MALDI-TOF DUB assay shows high sensitivity. Zoomed area (8,520–8,720m/z) of MALDI-TOF MS spectra for ubiquitin (Ubi) and15N-ubiquitin, in the presence of K11-linked diubiquitin are depicted. The limit of detection was determined as 2 fmol of ubiquitin on the target (in the presence of 42 fmol of15N-ubiquitin and 146 fmol of K11-linked diubiquitin). Presence of the doubly charged diubiquitin (diubiquitin [M+2H]2+) does not compromise identification of the singly charged ubiquitin (see alsoSupplementary Fig. 2). (c) Linearity and reproducibility of the MALDI-TOF DUB assay. Scatter plot of different concentrations of ubiquitin (10–10,000 nM) shows high linearity over about three orders of magnitude. Interday reproducibility was very high (Supplementary Table 1). Error bars represent s.d. of measurements. a.u., arbitrary unit; intens., intensity. Figure 1: The MALDI-TOF DUB assay. ( a ) Workflow of the MALDI-TOF DUB assay. Each of the 42 DUBs was incubated with all eight diubiquitin isomers individually (M1, K6, K11, K27, K29, K33, K48 and K63) for 60 min at 30 °C. The reaction was stopped with 2% TFA and mixed 1:1 with 0.5 μM 15 N-ubiquitin which serves as an internal standard. Subsequently, the analyte is mixed with 2,5 DHAP matrix and spotted onto a 1,536 AnchorChip MALDI target (Bruker Daltonics). Data analysis is performed using FlexAnalysis (Bruker Daltonics). ( b ) The MALDI-TOF DUB assay shows high sensitivity. Zoomed area (8,520–8,720 m / z ) of MALDI-TOF MS spectra for ubiquitin (Ubi) and 15 N-ubiquitin, in the presence of K11-linked diubiquitin are depicted. The limit of detection was determined as 2 fmol of ubiquitin on the target (in the presence of 42 fmol of 15 N-ubiquitin and 146 fmol of K11-linked diubiquitin). Presence of the doubly charged diubiquitin (diubiquitin [M+2H] 2+ ) does not compromise identification of the singly charged ubiquitin (see also Supplementary Fig. 2 ). ( c ) Linearity and reproducibility of the MALDI-TOF DUB assay. Scatter plot of different concentrations of ubiquitin (10–10,000 nM) shows high linearity over about three orders of magnitude. Interday reproducibility was very high ( Supplementary Table 1 ). Error bars represent s.d. of measurements. a.u., arbitrary unit; intens., intensity. Full size image The high resolution and mass accuracy of this MALDI-TOF mass spectrometer enabled baseline-resolution of isotopic patterns of ubiquitin and thus reliable quantification of the area of the ubiquitin peak. Moreover, it permitted clear separation of the doubly charged diubiquitin molecule ( m / z 8,556.64) and the singly charged monoubiquitin ( m / z 8,565.76; Fig. 1b ; Supplementary Fig. 1 ). Next, we tested the linearity of our assay by analysing standard curves over the ubiquitin concentration range of 10–10,000 nM (2–2,000 fmol on target) in the presence of 250 nM 15 N-Ubiquitin (42 fmol on the target) and 874 nM diubiquitin (15 ng μl −1 ; 146 fmol on the target) in three separately performed experiments on different days. Addition of 15 N-ubiquitin and/or diubiquitin isomers, did not affect sensitivity with which ubiquitin could be detected and quantified ( Supplementary Fig. 2 ). Average correlation coefficient ( r 2 ) for the three curves was not less than 0.99 ( Fig. 1c ) showing high linearity over a range of more than 500 ( Supplementary Table 1 ). The mean intraday precision and interday accuracy for ubiquitin/ 15 N-ubiquitin were 8% and 10%, respectively, demonstrating the suitability of the assay as a screening tool. The lower limit of quantification, defined as the lowest concentration that could be measured with a precision and accuracy better than 20%, was 10 nM (2 fmol on target; Fig. 1b ) allowing for significantly reduced enzyme and substrate amounts compared with previously used low-throughput methods that typically employed up to 4 μg of diubiquitin (234,000 fmol) per assay. Determining DUB specificity Utilizing the MALDI-TOF DUB assay, we systematically assessed the specificities of 42 recombinant human DUBs ( Table 1 ) against all possible ubiquitin chain linkages. This represents almost 50% of the DUBs encoded in the human genome. For this, we determined the DUB activity at five different enzyme concentrations (from 0.02 to 200 ng μl −1 ) against M1/linear, K6, K11, K27, K29, K33, K48 and K63-linked diubiquitin isomers, all at a final concentration of 1.46 μM in the assay. Altogether we performed more than 5,520 enzymatic reactions, providing the largest published resource for DUB specificity and activity ( Fig. 2 ). The results of this analysis highlighted a striking linkage specificity for five human DUBs (OTULIN—M1/linear, OTUB1—K48, AMSH, AMSH-LP and BRCC3—K63), which cleaved only one diubiquitin substrate even at very high concentrations of enzymes ( Fig. 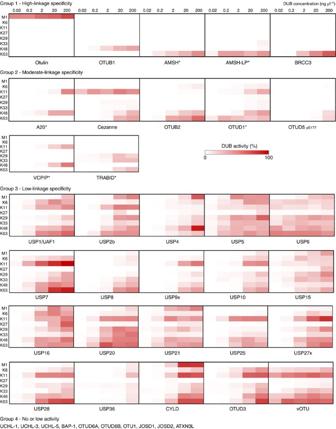Figure 2: Characterizing the linkage specificity of DUBs. Increasing concentrations (0.02–200 ng μl−1) of DUBs were incubated in triplicate with 1.46 μM of diubiquitin of each linkage type (M1, K6, K11, K29, K33, K48, K63 from Boston Biochem, K27 in-house produced) for 60 min at 30 °C and analysed by the MALDI-TOF DUB assay. The amount of monoubiquitin formed by this reaction was determined by MALDI-TOF MS and used to establish the DUB activity for individual diubiquitin isomers which is shown in a gradient of white (0%) to dark red (100%). The data show that DUBs can be grouped into enzymes cleaving specifically one linkage type (group 1), few linkage types (group 2), unspecific (group 3) or inactive enzymes (group 4). For DUB characterization, seeSupplementary Figs 3 and 8. 2 , group 1), which is consistent with previous data analysing these enzymes [36] , [37] , [38] ( Supplementary Table 2 ). Group 2 consisted of three DUBs that were highly specific to one linkage at only low concentrations (Cezanne-K11, OTUD1-K63 and A20-K48) and four DUBs (TRABID-K29/K33, VCPIPcat-K11/K48, OTUB2- and phosphorylated OTUD5-K48/K63) that displayed moderate selectivity hydrolysing two ubiquitin linkages at low concentrations but were less selective at high concentrations ( Fig. 2 , group 2). Twenty DUBs, including all the active USP family members tested displayed little selectivity ( Fig. 2 , group 3), agreeing with previously reported findings [39] . Four DUBs showed only very low activity (OTUD6A, OTU1, JOSD2 and ATXN3L) and six DUBs including OTU6B, JOSD1, and all the ubiquitin C-terminal hydrolases (UCH) were inactive in our assay ( Fig. 2 , group 4; Supplementary Fig. 3 ). Table 1 DUB enzymes analysed in this study. Full size table Figure 2: Characterizing the linkage specificity of DUBs. Increasing concentrations (0.02–200 ng μl −1 ) of DUBs were incubated in triplicate with 1.46 μM of diubiquitin of each linkage type (M1, K6, K11, K29, K33, K48, K63 from Boston Biochem, K27 in-house produced) for 60 min at 30 °C and analysed by the MALDI-TOF DUB assay. The amount of monoubiquitin formed by this reaction was determined by MALDI-TOF MS and used to establish the DUB activity for individual diubiquitin isomers which is shown in a gradient of white (0%) to dark red (100%). The data show that DUBs can be grouped into enzymes cleaving specifically one linkage type (group 1), few linkage types (group 2), unspecific (group 3) or inactive enzymes (group 4). For DUB characterization, see Supplementary Figs 3 and 8 . Full size image In parallel, we also performed DUB fluorogenic Ubiquitin-Rhodamine110-Glycine activity assays ( Table 1 ) which are frequently used in the field [28] , [40] , [41] . We calculated the specific activity of each DUB in this assay and grouped these into four categories (very low, low, moderate and high activity). Interestingly, when we compared the MALDI-TOF DUB assay data with fluorescent assay data ( Table 1 ) we found 10 enzymes (USP9x, USP27x, USP36, CYLD, Otulin, OTUB1, OTUB2, AMSH, AMSH-LP and BRCC3) that were active only in the MALDI-TOF DUB assay. Four enzymes (USP10, USP28, A20 and VCPIP) displaying low activity in the fluorescence assay were significantly more active in the MALDI-TOF DUB assay. The majority (18 out of 42) of DUBs tested was active in the MALDI-TOF DUB assay and displayed moderate or high activity in the fluorescence assay. In contrast, seven DUBs including all members of the UCH family as well as OTUD6A, JOSD1 and JOSD2 were active in the Rhodamine assay but not in the MALDI-TOF DUB assay. We found that three DUBs tested (OTUD6B, OTU1 and ATXN3L) displayed very low or no activity, but nevertheless reacted with an active site-directed probe (C-terminal propargylated ubiquitin [42] ; Supplementary Fig. 4 ). Assessing potency and selectivity of DUB inhibitors We next evaluated whether the MALDI-TOF DUB assay had potential to be deployed to assess potency and selectivity of DUB inhibitors. To undertake this, we set up a panel of 32 DUBs each assayed with the preferred diubiquitin isomers displaying the highest specific activity at the lowest concentration ( Supplementary Fig. 3 ). As proof of concept, we screened nine previously reported DUB inhibitors and inhibitor candidates (compound 16 (ref. 43 ), L434078, WP1130 (ref. 44 ), P22077 (ref. 45 ), Febuxostat (ref. 46 ), SJB3-019A (ref. 47 ), PR-619 (ref. 45 ), HBX 41,108 (ref. 48 ), pimozide (ref. 41 )) as well as two E2/E3 ligase inhibitors that have potential to alkylate Cys residues (NSC 697923 (ref. 49 ) and BAY 11-7082 (ref. 50 )) at two concentrations against a group of 32 highly active DUBs from our assay ( Fig. 3 ; Supplementary Fig. 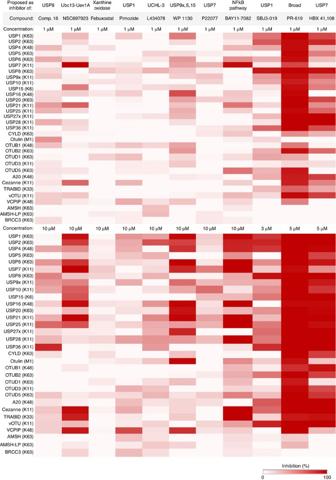Figure 3: Inhibition profiles of 11 DUB inhibitors and inhibitor candidates. Eleven different DUB inhibitors and inhibitor candidates were pre-incubated for 35 min at two different concentrations in duplicate (that is, two different experiments) with a panel of 32 DUBs and subsequently the specific substrate was added and incubated for 60 min (30 °C). Inhibition rates are colour coded with strongest inhibition in dark red, the diubiquitin topoisomers used for each DUB are in brackets. BAY 11-7082, NSC 697923 and SJB3-019A show some selectivity at 1 μM against USP7 and USP8, respectively, while PR-619 and HBX 41,108 inhibit strongly a wide range of DUBs even at low concentration. Other proposed inhibitors such as compound 16, L434078, WP1130 and P22077 show low activity and selectivity in this panel. 5 ; Supplementary Table 3 ). In addition, we performed IC 50 measurements for the DUBs that were most potently inhibited ( Fig. 4 ). For these studies, conditions were carefully optimized to ensure that assays were linear with respect to time ( Supplementary Fig. 6 ), and the diubiquitin substrate that displayed highest activity at the lowest DUB concentration was selected ( Supplementary Fig. 3 ). Figure 3: Inhibition profiles of 11 DUB inhibitors and inhibitor candidates. Eleven different DUB inhibitors and inhibitor candidates were pre-incubated for 35 min at two different concentrations in duplicate (that is, two different experiments) with a panel of 32 DUBs and subsequently the specific substrate was added and incubated for 60 min (30 °C). Inhibition rates are colour coded with strongest inhibition in dark red, the diubiquitin topoisomers used for each DUB are in brackets. BAY 11-7082, NSC 697923 and SJB3-019A show some selectivity at 1 μM against USP7 and USP8, respectively, while PR-619 and HBX 41,108 inhibit strongly a wide range of DUBs even at low concentration. Other proposed inhibitors such as compound 16, L434078, WP1130 and P22077 show low activity and selectivity in this panel. 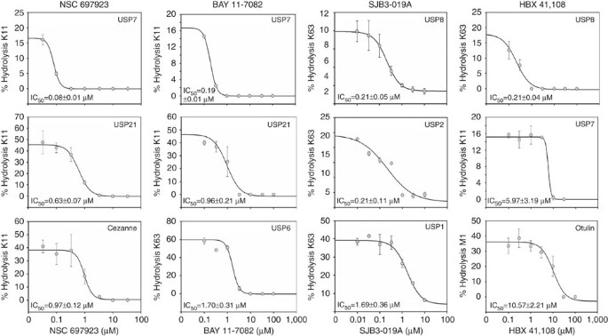Figure 4: IC50analyses of four inhibitors for selected DUBs. A subset of four inhibitors was chosen to characterize in more detail by determining their IC50for three DUBs. BAY 11-7082, NSC 697923 and SJB3-019A were chosen as they have some selectivity for one DUB, HBX 41,108 was chosen as it has been proposed as a USP7 inhibitor which is an attractive drug target51. Small inhibitor compounds were pre-incubated for 35 min at different concentrations (0–30 or 0–100 μM) in triplicates (that is, three different experiments) and subsequently the specific substrate was added and incubated for 60 min (30 °C). Diubiquitin topoisomers used for each DUB are named on theyaxis. Data show that NSC 697923 and BAY 11-7082 inhibit strongly USP7 with IC50<0.2 μM, while HBX 41,108 inhibits it at ~6 μM. SJB3-019A inhibits USP8 and USP2 about 10-fold better than USP1. See alsoSupplementary Table 4forPvalues. Error bars represent s.d. of measurements. For statistical analysis, four parameter logistic curve (best‐fit solution, nonlinear regression-dynamic fitting) and normality tests (Kolmogorov–Smirnov) are used (SigmaPlot, v. 12.5). Full size image Figure 4: IC 50 analyses of four inhibitors for selected DUBs. A subset of four inhibitors was chosen to characterize in more detail by determining their IC 50 for three DUBs. BAY 11-7082, NSC 697923 and SJB3-019A were chosen as they have some selectivity for one DUB, HBX 41,108 was chosen as it has been proposed as a USP7 inhibitor which is an attractive drug target [51] . Small inhibitor compounds were pre-incubated for 35 min at different concentrations (0–30 or 0–100 μM) in triplicates (that is, three different experiments) and subsequently the specific substrate was added and incubated for 60 min (30 °C). Diubiquitin topoisomers used for each DUB are named on the y axis. Data show that NSC 697923 and BAY 11-7082 inhibit strongly USP7 with IC 50 <0.2 μM, while HBX 41,108 inhibits it at ~6 μM. SJB3-019A inhibits USP8 and USP2 about 10-fold better than USP1. See also Supplementary Table 4 for P values. Error bars represent s.d. of measurements. For statistical analysis, four parameter logistic curve (best‐fit solution, nonlinear regression-dynamic fitting) and normality tests (Kolmogorov–Smirnov) are used (SigmaPlot, v. 12.5). Full size image Overall, none of the compounds tested displayed strong selectivity towards a single DUB and many were unselectively inhibiting most DUBs on the panel ( Fig. 3 ). For example, PR-619 (ref. 45 ; Supplementary Fig. 5Q,R ), is an ubiquitin/UbL isopeptidase inhibitor, which has previously been reported to inhibit a range of cysteine protease DUBs [45] . Consistent with this, we found that PR-619 inhibited 27 of the 32 tested DUBs with only members of the OTU and JAMM family being unaffected, likely because the latter are zinc- metalloproteases and do not possess a reactive catalytic Cys residue. Furthermore, our data indicate that SJB3-019A ( Supplementary Fig. 5O,P ), which has previously been shown to inhibit USP1 in leukaemic cells [47] , inhibits USP8 more strongly (IC 50 0.21 μM) than USP1 (IC 50 1.69 μM) but in addition also significantly inhibited several other DUBs tested. Another reported USP1 inhibitor, pimozide [41] , was also found to be nonselective, inhibiting many other DUBs with similar affinity to USP1 ( Supplementary Fig. 5E,F ). USP7 is one of the most targeted DUBs as phenotypes associated with USP7 silencing strongly suggest that small molecule inhibitors of USP7 may have the potential for antiviral and anticancer therapies [13] , [51] . HBX 41,108, a cyano-indenopyrazine inhibitor of USP7 that has been shown to stabilize polyubiquitylated p53 at high concentrations in HEK293 cells [48] inhibited 25 of the 32 DUBs tested more than 70% at 5 μM ( Fig. 3 ). This is consistent with another report suggesting that HBX 41,108 reacted with additional DUBs [52] . Only members of the JAMM family are not affected by HBX 41,108, again likely because they are zinc-metalloproteases and not cysteine proteases ( Supplementary Fig. 5S,T ). Out of the 11 compounds profiled, BAY 11-7082 and NSC 697923 both of which contain vinyl sulphone reactive groups ( Supplementary Table 3 ) were found to inhibit USP7 with moderate higher potency than other DUBs tested. For example, BAY 11-7082 and NSC 697923 inhibited USP7 with an IC 50 of 0.19 μM and 0.08 μM, respectively. The next most potently inhibited DUB, that is, USP21, was inhibited by BAY 11-7082 and NSC 697923 with an IC 50 of 0.96 μM and 0.63 μM, respectively. The potency of NSC 697923 for USP7 (0.08 μM) was 70-fold higher than that of HBX 41,108 (5.97 μM). We have developed a sensitive, reproducible and robust assay for the analysis of DUB in vitro activity and specificity. For this, we have made use of highly sensitive and fast MALDI-TOF mass spectrometry, which, due to the use of 1,536-sample targets, is suitable for robotic automation and thus high-throughput screening [53] . We circumvented spot-to-spot and shot-to-shot irreproducibility in MALDI ionization by using isotopically labelled ubiquitin as an internal standard as it guarantees identical extraction, crystallization and gas-phase behaviour. Overall, this setup allowed us to achieve very high precision, accuracy and linearity of measurements over concentrations of almost three orders of magnitude. The advantages compared with the commonly used assays with fluorogenic ubiquitin substrates are the use of substrates which are more physiological and the ability to analyse chain linkage specificity. Moreover, compared with current techniques using SDS–PAGE, our assay is considerably faster (2–4 h for the acquisition of 1,536 data points) and more sensitive, thus requiring vastly reduced amounts of diubiquitin substrate. It should be noted that the assay is currently pipetted manually and due to addition of matrix and trifluoroacetic acid (TFA), only 3.3% of the initial reaction mixture is utilized for the mass spectrometry analysis. Thus, after optimization, it should be feasible to scale down reaction amounts at least another 20-fold using nanoliter dispensing robotics representing a nearly 600-fold reduction in amounts of diubiquitin needed in current low-throughput assays. Our data has established that the MALDI-TOF DUB assay is a powerful approach to define the substrate specificity of DUBs. Using only 120 data points we have devised a strategy to characterize the activity of each DUB in triplicate (that is, three different experiments) over five concentrations spanning 10,000-fold range against all eight diubiquitin chain linkages. Only a few of the 42 expressed DUBs, and here particularly the members of the UCH family, were inactive in the MALDI-TOF DUB assay but showed high activity in the fluorogenic Ubiquitin-Rhodamine110-Glycine assay ( Table 1 ). This is consistent with previous work which has shown that UCH DUBs cleave ubiquitin moieties from protein substrates but do not hydrolyse diubiquitin [45] , [54] . Interestingly, we found that members of the JAMM family (AMSH, AMSH-LP and BRCC3) displayed high activity in the MALDI-TOF DUB assay, exhibiting exquisite preference for K63 linkages, but were completely inactive in the fluorescence Ubiquitin-Rhodamine110-Glycine assay ( Table 1 ). Therefore the MALDI-TOF DUB assay is the preferred technology to undertake future screening for specific inhibitors that target these metalloproteases. Among the other inactive DUBs are ATXN3L (MJD+ family DUB) that has been shown to preferentially cleave ubiquitin chains with more than four units [30] , which is likely to explain why no activity was observed in the MALDI-TOF DUB and Ubiquitin-Rhodamine110-Glycine assays. Furthermore, OTUD6B was also previously shown to be inactive against ubiquitin dimers using a low-throughput assay [37] . In our hands, full-length OTU1 expressed in Escherichia coli ( E. coli ) only displayed trace activity towards K11, K48 and K63 at the highest concentration tested (200 ng μl −1 ; 3.1 μM). In another study full-length OTU1 assayed at 4 μM was shown to display low activity against K11, K27, K29, K33 and K48 (ref. 37 ). A different group has suggested that OTU1 preferentially hydrolyses longer polyubiquitin chains [55] , which might explain the weak activity observed [55] . Further work is also required to assess whether the other enzymes might require cofactors or posttranslational modifications, such as phosphorylation for optimal activity as reported for OTUD5 (ref. 56 ). In the future, we intend to increase the coverage of the DUB family by including more enzymes. These proteins will be also expressed in either bacterial or insect cultures and if the full-length protein cannot be purified, a shorter construct encompassing the catalytic domain will be expressed. Our data compare well to very recently published data of DUBs of the OTU family [37] , confirming high specificity for many members of this family. Also other DUB families, such as the unspecific USPs as well as the specific JAMMs are in agreement with the published data [38] , [39] ( Supplementary Table 2 ). Yet, our data also suggests that the specificity of several DUBs depends on the concentration of the enzymes and the enzyme/substrate ratio. In general, highest selectivity is observed at low concentrations of DUBs. Cezanne for example, is very active and specific for K11 at the lowest concentration tested (that is, 0.02 ng μl −1 ; ~0.2 nM). Similarly, OTUD1 is very selective for K63 at 0.2 ng μl −1 (~5 nM). However, at higher concentrations, both Cezanne and OTUD1 lose their specificity. These observations highlight that these enzymes are not completely selective and possess the ability to weakly act on other topoisomers at higher substrate concentrations. Even several USPs, which are mostly unspecific in our assay, present some specificity at the lowest concentrations analysed. This emphasizes the importance that specificity of DUBs should be tested over a wide range of enzyme concentrations, which has not generally been undertaken in previous analyses. The consistency of our data compared with previous work on DUB activity and selectivity highlights the reliability of the MALDI-TOF DUB assay technology. None of the DUBs tested initially displayed significant activity against K27-linked diubiquitin isomers that were purchased commercially. We confirmed by mass spectrometry that the commercial K27 diubiquitin molecule was indeed correctly linked and was present in equimolar amounts compared with the other diubiquitin isomers. We determined by pseudo-selected reaction monitoring (pSRM) against the linkage peptides that this diubiquitin contained small amounts (~7%) of K11 and (~8%) K63 diubiquitin chains, which were not affecting overall results though ( Supplementary Figs 10 and 11A ). In addition, we performed circular dichroism to rule out misfolding of the isomer ( Supplementary Fig. 11B ). However, to ensure that the inactivity of all DUBs against this linkage was not due to quality issues of the commercially produced K27 diubiquitin, we compared three differently sourced versions of K27 diubiquitin (Boston Biochem, UbiQ and in-house chemically engineered K27 diubiquitin [57] , [58] ) against four DUBs that had shown activity against K27 in previous publications [25] , [39] . While USP7, USP8 and USP25 could not hydrolyse any of the three differently sourced K27 diubiquitins in our hands, we observed that USP16 displayed strong activity against this linkage for in-house K27 diubiquitin but not for the commercially sourced K27-chains ( Supplementary Fig. 11C ). It should be noted that previous work [39] also concluded that USP16 displayed highest activity towards K27-linked diubiquitin isomers compared with the other DUBs tested, suggesting that this enzyme might indeed cleave this chain type in vitro . It is not clear why there is this discrepancy in activity of USP16 towards in-house chemically engineered (GOPAL methodology) and commercially available K27 diubiquitin. We therefore re-tested the whole DUB panel against the in-house K27 diubiquitin and except for USP16, no other DUB showed any significant activity, agreeing with the data obtained with commercially sourced K27 diubiquitin. This suggests that extra caution is required when K27 diubiquitin is used for DUB assays. There is a huge interest in developing chemical probes that target specific components of the ubiquitylation system [59] . We have shown that the MALDI-TOF DUB assay can be readily used to determine inhibition rates and the IC 50 of small molecule inhibitors of DUBs. The MALDI-TOF DUB assay also enables the facile profiling of inhibitors against numerous DUBs acting on a more physiological substrate than fluorescent ubiquitin conjugates that have been previously employed for this purpose [28] . Moreover, one will be able to employ this assay using other physiological substrates, such as ubiquitylated proteins. As proof of concept, we have deployed a panel of 32 active DUBs to profile 11 available DUB inhibitors and inhibitor candidates. Our work confirms previous work that PR-619 is a general DUB inhibitor that potently suppresses the activity of almost all cysteine protease DUBs [45] . Similarly HBX 41,108, proposed as an USP7 inhibitor [48] , inhibited almost all DUBs in our assay better than USP7. Out of the compounds analysed, BAY 11-7082 and NSC 697923 displayed the highest selectivity, inhibiting USP7 with five- to eightfold higher potency than the second most sensitive DUB on our panel (that is, USP21). BAY 11-7082 inhibits NFκB signalling [60] and was recently shown to inhibit the majority of E2 and E3 ligases tested by reacting covalently with the catalytic cysteine residues [50] . Moreover, BAY 11-7082 also inhibits several tyrosine phosphatases by reacting with catalytic Cys residue of these enzymes [61] . NSC 697923 was originally shown to inhibit the E2 ligase Ubc13-Uev1A [49] . These data suggest that BAY 11-7082 and NSC 697923 are likely to inhibit a broad range of enzymes possessing catalytic Cys residues. Nevertheless, the moderate specificity of these compounds for USP7 indicates that it might be possible to further engineer these compounds towards more selective probes. Furthermore, we could show that SJB3-019A and pimozide, two proposed USP1 inhibitors [41] , [47] , inhibit USP8 at a 10-fold lower concentration or showed poorly selectivity, respectively. Overall this data reveal the importance of undertaking extensive profiling of specificity of DUB inhibitors as it is essential to ensure the selectivity of these compounds for in vivo applications. To screen larger numbers of small molecule inhibitors, we propose a future screening strategy ( Supplementary Fig. 7 ) that can be summarized in three steps: screen 1, screening a large number of small molecules against a single DUB to identify lead candidates; screen 2, inhibitor specificity determination of these lead candidates at a single concentration against a panel of a large number of DUBs; screen 3, determination of IC 50 for best DUB/inhibitor pairs. We believe that such strategies will be useful for discovery of specific inhibitors of DUBs which have the potential to become important future drug targets [22] . In conclusion, we present here a novel screening method to assay DUB activity and specificity with high sensitivity, reproducibility and reliability, which is able to carry out precise quantified measurements at a rate of ~6–9 s per sample spot. Using physiological substrates of DUBs allowed us to determine specificity of 42 human DUBs among which several showed high specificity for one single-chain type. This data allowed us to generate a simple array of preferred chain types and lowest concentrations of activity for each DUB which will serve as a sensitive and fast tool for screening for DUB inhibitors. Materials Ubiquitin monomer, BSA, Tris and DTT were purchased from Sigma-Aldrich. Diubiquitin topoisomers (M1, K6, K11, K27, K29, K33, K48 and K63-linked) were purchased from Boston Biochem (Boston, MA), additional K27 diubiquitin was produced in-house [57] , [58] , whereas all MALDI-TOF MS materials (targets, matrix and protein calibration mixture) were purchased from Bruker Daltonics (Bremen, Germany). PR-619 and P22077 (Calbiochem/Merck, Darmstadt, Germany) as well as HBX 41,108, pimozide and degrasyn/WP1130 (Tocris Bioscience, Bristol, UK) and L434078 (Sigma-Aldrich, St Louis, MO, USA) were purchased commercially. Febuxostat, SJB3-019A, compound 16, NSC 697923 and BAY 11-7082 were synthesized ( Supplementary Table 3 ). Expression of DUB enzymes For bacterial expression, full-length or catalytic core domains for various DUB enzymes were cloned into either pET-24, pET-28 (Novagen) or pGEX6P (GE Healthcare) vectors to express either N-terminally tagged 6xHis or GST tagged proteins. Recombinant proteins were expressed in E. coli Bl21 (DE3) cells which were lysed by sonication lysis buffer (50 mM Tris–HCl pH 7.5, 250 mM NaCl, 0.5 mM EGTA, 0.5 mM EDTA, 0.5% Triton X-100, 1 mM DTT, 1mM Pefabloc, 10 μg ml −1 Leupeptin), then centrifuged to remove insoluble material. For protein purification, supernatants were subjected to affinity chromatography using either Ni 2+ -NTA-Sepharose (GE Healthcare) or Glutathione-Sepharose (Expedeon) resin. For insect cell protein expression, appropriate cDNAs were cloned into the pFastBac vector, baculoviruses were generated to encode various Dac-tagged [62] DUB enzymes. Sf21 cells were typically infected with P1 virus stocks and harvested 48 h later. Cells were lysed in Dac lysis buffer (40 mM Tris pH 7.5, 0.2% Triton X-100, 0.5 mM EGTA, 0.1 mM EDTA, 1mM DTT) supplemented with 1 mM Pefabloc and Leupeptin at 20 μg ml −1 , then centrifuged to remove insoluble material. For protein purification, supernatants were subjected to affinity chromatography using ampicillin-Sepharose resin for 45 min at ambient temperature. The DUB enzymes were either eluted from the ampicillin-Sepharose by incubating 4 × for 15 min with 1 resin volume of 50 mM Tris-HCl pH 7.5, 5% v/v glycerol, 100 mM NaCl, 10 mM ampicillin, 1 mM DTT, 0.03% (w/v) Brij-35 or recovered by digesting the DUB off the Dac-tag using TEV-protease in 50 mM Tris–HCl pH 7.5, 100 mM NaCl, 0.03% (w/v) Brij-35 ( Supplementary Fig. 8 ). 15 N-ubiquitin expression and purification Untagged full-length human ubiquitin was cloned into the pET-24 vector and expressed in E. coli Bl21 (DE3) cells. Cells expressing 15 N-ubiquitin were grown in M9 minimal media supplemented with 15 N ISOGRO (Sigma) and Ammonium- 15 N chloride (Sigma) according to the manufacturer’s instructions. Cells were sedimented, resuspended in H 2 O and lysed by freeze-thawing, then centrifuged to remove insoluble material. Bacterial proteins were precipitated by dropping the pH to 4.5 with diluted HClO 4 , then sedimented by centrifugation. The supernatant containing the ubiquitin was adjusted to 20 mM ammonium-acetate pH 4.5 and applied to a Source 15 S HR10/10 column (GE Healthcare), which was developed with a gradient of 0–1 M NaCl. The 15 N-ubiquitin eluting at a conductivity of 18 mS cm −1 was concentrated and subjected to chromatography on a Superdex75 XK16/60 column (Amersham). Final 15 N-ubiquitin fractions were pooled and concentrated to 35 mg ml −1 . MALDI-TOF MS analysis revealed a 97% incorporation of 15 N ( Supplementary Fig. 9 ). Preparation of K27-linked diubiquitin K27-linked diubiquitin was prepared as described [57] with the following exceptions. Acceptor ubiquitin was expressed from a new plasmid (pCDF-pylT-UbTAG27-His6) carrying an amber stop codon at residue position 27 of ubiquitin. Crude Cbz-deprotected ubiquitin species were then dissolved in denaturing buffer (200 mM Na 2 HPO 4 pH 7.5, 6 M guanidinium chloride) at a final concentration of ~2mg ml −1 . Deprotected diubiquitin was then purified from residual monoubiquitin by semi-preparative reversed-phase HPLC using a Dionex Ultimate 3000 system. A flow rate of 10 ml min −1 and a gradient of 20% solvent A to 50% solvent B over 40 min were used with a Thermo Biobasic C4 (250 mm × 21.2 mm) column (solvent A=0.1% trifluoroacetic acid in H 2 O; solvent B=0.1% trifluoroacetic acid in acetonitrile). Fractions corresponding to K27-linked diubiquitin were determined by liquid chromatography–MS and were then pooled and freeze dried. Freeze dried K27-linked diubiquitin was dissolved in denaturing buffer to a final concentration of 2 mg ml −1 and folded by overnight dialysis against PBS. In vitro DUB assays and inhibitor screening To monitor DUB activity in vitro , we tested a panel of 42 human DUBs at different concentrations (0.02-0.2-2-20-200 ng μl −1 ) against all diubiquitin topoisomers (M1, K6, K11, K27, K29, K33, K48 and K63-linked chains) as substrates at a fixed concentration (25 ng μl −1 , 1.46 μM). Both enzymes and substrates were freshly prepared in the reaction buffer (40 mM Tris–HCl, pH 7.6, 5 mM DTT, 0.005% BSA) for each run. The enzymes were pre-incubated in the reaction buffer for 10 min at 30 °C; afterwards, the diubiquitin isomers were added and the reaction mixture incubated for 60 min at 30 °C. The reaction was stopped by adding TFA to a final concentration of 2% (v/v). Possible background due to contamination of the diubiquitin with ubiquitin monomers was measured in a reaction buffer in which the enzyme was excluded and ubiquitin intensities normalized accordingly ( Supplementary Fig. 10B-2 ). Dimer purity was controlled by SDS–PAGE, PRM and MALDI-TOF MS/MS ( Supplementary Figs 10 and 11 ). For the small molecule inhibitor studies, we tested the MALDI-TOF DUB methodology by screening 11 DUB inhibitors or inhibitor candidates. To assess linearity for inhibitor experiments, time-dependent inhibition experiments were performed by adding increasing concentrations of the compound, from 0 to 90 μM, to the reaction buffer containing USP7 (1 ng μl −1 ) and incubated for 30 min at 30 °C. We demonstrated the linearity of response of USP7 (1 ng μl −1 ) versus K11-linked diubiquitin (1.46 μM) to increasing concentrations of PR-619 (0–40 μM) over time (0–20 min) ( Supplementary Fig. 6 ). Some of these inhibitors could potentially react with reducing agents present in the assay such as dithiothreitol (DTT) or tris(2-carboxyethyl) phosphine (TCEP). We therefore verified using MALDI-TOF mass spectrometry whether the inhibitor compounds reacted with either 1 mM DTT or 0.5 mM TCEP when incubated at 30 °C for 1 h under the DUB assay conditions employed. This revealed that only WP1130 significantly reacted with both DTT and TCEP under these conditions (data not shown). For all inhibitor experiments, except PR-619 and HBX 41,108, no DTT but the remaining trace levels from the protein expression was added to the reaction buffer. Following the scheme in Supplementary Fig. 7 , we determined the activity of the inhibitors in two steps. First of all, we screened the inhibitors in duplicates against 32 DUBs. The enzymes were pre-incubated with either 1 or 3/5/10 μM of inhibitor for 35 min at 30 °C. Next, substrates were incubated with the enzyme plus inhibitor mixture for 60 min at 30 °C. Second, we determined the inhibitors’ IC 50 on a subset of selected DUBs. For calculation of IC 50 , data were fitted in SigmaPlot (v. 12.5 Build 12.5.0.38) using the four parameter logistic equation: y =min+(max−min)/( x /IC 50 ) Hillslope. Values of IC 50 for all compounds are summarized in Supplementary Table 4 . Analysis by MALDI-TOF MS Sample preparation. Acidified samples of the DUB assays were mixed with 0.5 μM 15 N-ubiquitin and then with one part of 2% (v/v) TFA and one part of 2,5 DHAP matrix solution (7.6 mg of 2,5 DHAP in 375 μl ethanol and 125 μl of an aqueous 12 mg ml −1 diammonium hydrogen citrate). Then 0.5 μl of these solutions were spotted in replicates onto an MTP AnchorChip 1,536 TF (600 μm anchor, Bruker Daltonics). Data acquisition. A high resolution MALDI-TOF MS instrument (UltrafleXtreme, Bruker Daltonics) with Compass 1.3 control and processing software was used. Samples were run in automatic mode (AutoXecute, Bruker Daltonics) allowing 6–9 seconds per spot, using the 1,536 spots AnchorChip. Ionization was achieved by a 1-kHz smartbeam-II solid state laser with a fixed initial laser power of 60% (laser attenuator offset 68%, range 30%) and detected by the FlashDetector at detector gain of × 10. Reflector mode was used with optimized voltages for reflector-1 (26.61 kV) and reflector-2 (13.39 kV), ion sources (IonSource-1: 24.86 kV, IonSource-2: 22.71 kV) and pulsed ion extraction (320 ns). Sampling rate was 0.25 ns equivalent to a 4 GS/s digitization rate. An amount of 2,100 (3 × 700) shots were summed up in ‘random walk’ and with ‘large’ smartbeam laser focus. Spectra were accumulated by FlexControl software (v. 3.3 Build 108), processed using FlexAnalysis software (v. 3.3, Build 80) and the sophisticated numerical annotation procedure (‘SNAP’) peak detection algorithm, setting the signal-to-noise threshold at 250. Before calibration, the spectra were processed using smoothing (Savitzky–Golay algorithm) and baseline subtraction (‘TopHat’) for reproducible peak annotation on nonresolved isotope distributions: one cycle, 0.2 m / z for the width. For external interactive calibration in quadratic mode, the ‘Protein Calibration Standard 1’ (Bruker) was used with ubiquitin ([M+H] + average=8,565.76), myoglobin ([M+2H] 2+ average=8,476.66) and cytochrome c ([M+2H] 2+ average= 6,181.05, [M+H] + =12,360.97) ions as average m / z values. Internal calibration was performed using the ubiquitin peak ([M+H] + average=8,565.76). An example of a full scan MALDI spectrum is depicted in Supplementary Fig. 12 . Data analysis. A modified method for data acquisition was developed for FlexAnalysis Software, using the SNAP algorithm. This algorithm is calculating an isotopic distribution which best fits the pattern of an isotopically resolved protein signal. For area calculation, the complete isotopic distribution was taken into account. Data output was exported as a. csv file using FlexAnalysis Batch Process (Compass 1.3) and further processed in Microsoft Excel, where plotting of graphs, calculation of s.d. and coefficient of variation (%) were performed. The measurement of DUB activity (% of diubiquitin isomer consumed, x ) from relative isotopic distribution summed area ratios was performed according to equation (1), Quality control of diubiquitin isomers by MALDI-TOF and PRM Two micrograms of each diubiquitin chain was resolved by SDS–PAGE (4–20%, Tris-Glycine, Novex, Life Technologies), stained by InstantBlue Coomassie stain (Expedeon). Bands were excised and digested with trypsin ( Supplementary Fig. 10A ). Gel pieces were washed subsequently with water, 50% methanol/water, 0.1 M NH 4 HCO 3 , then shrunk in acetonitrile and digested with trypsin (Pierce). The digestion was performed overnight at 37 °C and peptides were extracted further in 50% acetonitrile/2.5% TFA. Digests were dried and reconstituted in 0.1% TFA/water to 15 μg ml −1 . A total of 30 ng of each digest was injected onto a 15 cm × 75 μm (I.D.) EasySpray column (Thermo Fisher Scientific) and analysed on an LTQ-Velos Pro ion trap (Thermo Fisher Scientific) using a PRM [63] specific for each diubiquitin chain linkage (Gly-Gly) peptide ( Supplementary Figs 10C and 11A ). Lists of precursor masses and fragment transitions are reported in Supplementary Table 5 . Data were acquired in a data-independent mode with one full scan followed by 10 MS 2 scans with the masses of the different linkages. MS 2 occurred even if precursor mass was not detected in MS 1 scan. Extracted ion chromatograms of the MS 2 spectra for each diubiquitin chain peptide was performed by summing the ion current of the three or four most dominant daughter ions. The linkage peptide of K29-diubiquitin does not bind to the trap column (Acclaim PepMap100 C18, 5 μm, Thermo Fisher Scientific) of the liquid chromatography–MS system under normal conditions. We therefore analysed the purity of this diubiquitin by MALDI-TOF MS ( Supplementary Fig. 10D ). Fifteen nanograms per microlitre of digested diubiquitin was mixed with 10 mg ml −1 alpha -cyano-4-hydroxycinnamic acid (1:1) and spotted onto a 384 AnchorChip target (Bruker Daltonics). For MS 2 , LIFT technology was performed and the data were processed by Mascot server through BioTools (Bruker Daltonics). Ubiquitin-Rhodamine110-Glycine expression, purification and preparation For the cloning of the ubiquitin-intein-His 6 expression vector, the coding region for amino acids 1–75 of human ubiquitin were amplified by PCR with suitable primers for subsequent cloning into intein expression vector pTYB2 as described [28] . Ubiquitin-intein-His 6 was expressed and purified as described [28] with the following exceptions. Ubiquitin-intein was batch purified on nickel chelating affinity media (Amersham) and Ubiquitin-MES was released by addition of 100 mM Na-mercaptoethanesulfonate (MES) for 5 h at 22 °C. Ubiquitin-MES was eluted with 4 column volumes of 20 mM 2-(N-morpholino) ethanesulfonic acid, pH 6.5, 100 mM NaCl. Eluted material was concentrated by ultrafiltration (Vivaspin 6, 5-kDa cutoff) to <5 ml and supplemented with 10 eq. N-hydroxysuccinimide (Fluka 56480), 10 eq. sym-collidine (Fluka 27690) and 15 eq. bis-glycyl-rhodamine110 (prepared in-house) for 24 h at 37 °C. For purification the reaction mixture was desalted into 20 mM 2-(N-morpholino) ethanesulfonic acid, pH 6.5 on a HiPrep Sephadex G-25 26/10 column (GE healthcare) then applied to a Source 15 S HR 10/10 column (GE healthcare) which was developed with a gradient of 0–1 NaCl. Final Ubiquitin-Rhodamine110-Gly fractions were pooled, dialysed into 50 mM Tris, pH 7.5 then concentrated to 1 mg ml −1 . In the fluorescent assay, 0.5 μM Ubiquitin-Rhodamine110-Gly in 40 mM Tris-HCl buffer, pH 7.6, 5 mM DTT and 0.05 mg ml-1 BSA were incubated with 0.05–5 ng μl −1 of each DUB for 60 min at 30°C. Samples were prepared in triplicates and analyzed in 96-well plates using a Perkin Elmer Envision 2104 multi label reader at Excitation/Emission 485/535 nm (ref. 28 ). How to cite this article: Ritorto, M. S. et al . Screening of DUB activity and specificity by MALDI-TOF mass spectrometry. Nat. Commun. 5:4763 doi: 10.1038/ncomms5763 (2014).